Increasing our ability to predict contemporary evolution Prediction is a core component of the sciences. However, evolutionary biology is often portrayed as a descriptive or historical science, rather than a predictive one [1] , [2] , [3] . Nonetheless, the predictability of evolution can be quantified, for example by testing how well existing time series predict future evolutionary changes (Fig. 1 ) [1] , [4] . Besides its scientific importance, our ability to predict evolution has applied implications, for example for the development of vaccines and antibiotics (i.e., viruses and bacteria evolve to be resistant), animal breeding programs aimed at conservation and reintroduction, and biocontrol of insect pests that attack crops and lumber. Fig. 1: Quantifying the predictability of short-term evolution using time-series data. Autoregressive moving average (ARMA) models can be applied to existing data to generate predictions for future trait values or allele frequencies. In turn, the fit (e.g., r 2 value) of these predicted values to those actually observed provides a metric of the predictability of evolution. Full size image Here we focus on predictability defined as the ability to forecast future trait values or allele frequencies using existing data (Fig. 1 ). Such predictive ability can be studied using temporal data alone, or by adding information on the mechanisms and genomic basis of evolution [5] . We focus on contemporary evolution using time-series data spanning several to dozens of generations (i.e., in many organisms this will equate to decades), where evolution may proceed via standing genetic variation or new mutations. This focus on medium-term evolution complements quantitative genetics work on the predictability of immediate, single-generation responses to selection and studies that consider parallel and repeated evolution over longer (e.g., phylogenetic) time scales [3] , [6] . The degree to which evolution is predictable forms a long-standing debate in biology [3] , [7] . At the core of this debate is the question of the extent to which evolution is driven by random versus deterministic processes [3] (Fig. 2 ). In this context, there are two main classes of explanation for difficulties in predicting evolution. First, predictability can be limited by random processes (the “random limits” hypothesis) [8] . The key mechanisms underlying this hypothesis are stochastic changes in allele frequency due to genetic drift and the random nature of mutation. Second, even evolution driven by deterministic natural selection can be difficult to predict, due to limited data that in turn leads to poor understanding of selection and its environmental causes, trait variation, and inheritance [4] , [9] , [10] (the “data limits” hypothesis). Indeed, a starting point for improving our ability to predict evolution is to increase understanding of when selection is expected to be directional, fluctuating, or stabilizing. Fig. 2: Schematic illustration of two hypotheses for limitations on predicting evolution. This includes depiction of the evolutionary processes involved, and data which might be used to improve prediction. QTL quantitative trait locus, GWA genome wide association. Full size image These explanations are not mutually exclusive and are likely to operate simultaneously. However, they are conceptually distinct due to core differences in the factors that they propose to limit our ability to make accurate predictions; inherent unpredictability caused by stochastic processes underlies the random limits hypothesis, whereas insufficient knowledge on the part of those trying to form predictions underlies the data limits hypothesis. In terms of the data limits hypothesis, the underlying assumption is that with sufficient data and proper analysis, deterministic processes can be predicted. Thus, shortcomings in predictive ability stem largely from insufficient data and inadequate analytical tools, not from inherent randomness per se. Limits to data and our understanding of evolutionary process can arise at several levels. First, the environmental sources of selection, such as climatic conditions or predator abundance, might fluctuate in ways that are themselves difficult to predict, even if they are deterministic [1] . We stress that even deterministic environmental fluctuations might appear random, due to sensitivity to initial conditions that generates chaotic dynamics [11] . Such chaotic fluctuations are not truly random and our ability to predict them is still, in principle, tied to data limits. Second, even if environmental changes can be predicted, poor understanding of how environmental factors affect resource distributions and impose selection on phenotypes can reduce predictive ability for trait evolution. Third, poor understanding of the genetic architecture of traits can produce difficulties predicting genetic change from patterns of phenotypic selection [5] , [12] . For example, prediction can be complicated by phenotypic plasticity, which may be a common way that organisms respond to environmental change [13] . At all these levels, limits can arise in the quality or quantity of data, and in analysis. Such data limits are exacerbated by the potential for different factors to act at varying temporal and spatial scales, and by the fact that rare and difficult to predict environmental changes can have large effects on evolution. These general concepts apply across environmental factors, traits, and taxa, as outlined in Box 1 using examples in birds, insects, and other organisms. Box 1. Examples of our ability to predict evolution in natural populations We here discuss progress and challenges in predicting evolution using empirical examples. A first example involves fluctuating selection caused by climatic variability, which has been documented in numerous species [26] , [27] , [28] ; (Fig. 3a ). Perhaps the best example stems from long-term studies of beak size evolution in Darwin’s finches [1] . Here, variation in rainfall on Daphne Major has been shown to affect the relative abundances of small versus large seeds, which in turn can exert selection on beak size in Geospiza fortis during drought conditions. Thus, rare and difficult-to-predict droughts can have large effects on evolution. Indeed, in the case of G. fortis it could be argued that evolution is unpredictable not because we don’t understand selection (i.e., selection is known to be exerted by seed size distributions), but rather because available data and models cannot predict climatic fluctuations, or how these affect seed size distributions. Thus, prediction in this case was limited ( r 2 ~ 0.14, this value is a point estimate from autocorrelation analysis of how well trait values for beaks in the past predict those in the future, see also Fig. 1 ) [4] , and might be improved via better climate models and data on how climate affects resource distributions. A second example involves predation, which is a common source of natural selection that can fluctuate according to prey characteristics (Fig. 3b ). In particular, predation can cause negative frequency-dependent selection (NFDS) when predators focus on more common prey types. In such cases, the fitness of a phenotype fluctuates because it depends on the phenotype’s frequency in the population, and is higher when the phenotype is rare. This has been documented, for example, in cichlids, guppies, stickleback, and stick insects [4] , [29] , [30] , [31] . Such systems represent cases where evolution is expected to be easier to predict. Even with NFDS, however, data limits can apply, as illustrated by long-term studies of the evolution of striped and unstriped cryptic color morphs in Timema cristinae stick insects [4] . In T. cristinae , morph frequencies fluctuate predictably among years ( r 2 ~ 0.90) and there is experimental support for NFDS. Specifically, an experiment showed that the striped morph is strongly favored when initially rare (i.e., 20% initial frequency), but shows idiosyncratic changes when initially common (80% initial frequency). Whether selection would differ if ratios were manipulated more extremely is unclear. Moreover, why fluctuations occur at yearly, rather than monthly, scales is unknown. Thus, prediction might be improved by estimating the quantitative form of the NFDS fitness function, and via understanding factors that affect the foraging behavior and search images of bird predators. Nonetheless, evolution was highly predictable in this example, and the mechanisms of evolution are reasonably understood due to insights from combining experiments and genomics. Specifically, experiments support NFDS and genomic data rule out a predominant role for random genetic drift, and have clarified the role of epistasis [32] and suppressed recombination in the evolution of color genes. The examples in Box 1 illustrate how data limits in even well-studied systems can mediate the extent to which scientists can predict evolution. However, rather than dampening hope for prediction, the results suggest that progress can be made with empirical effort, for example via coupling long-term monitoring of populations with large, replicated experiments that reveal evolutionary process, and powerful genomic tools that allow dissection of the genetic basis of traits. Nonetheless, gathering such data will rarely be a trivial task. At a minimum, obtaining time-series data necessarily takes time, and this cannot be sped up with more effort. Identifying and measuring additional factors affecting evolutionary dynamics, such as relevant environmental parameters and selection estimates, increases the effort required. Simulation models calibrated based on empirical understanding of a system may aid in parsing the effects of different factors on predictability (e.g., variation in selection, genetic architecture, random drift), thus guiding researchers as to where further effort is best placed, the sample sizes required to increase precision, etc. 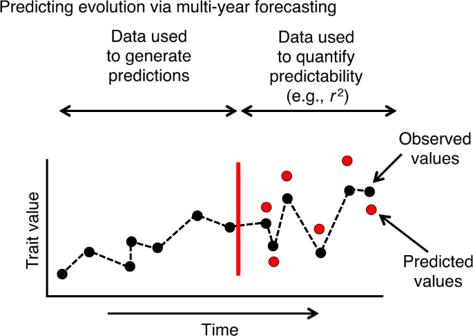Fig. 1: Quantifying the predictability of short-term evolution using time-series data. Autoregressive moving average (ARMA) models can be applied to existing data to generate predictions for future trait values or allele frequencies. In turn, the fit (e.g.,r2value) of these predicted values to those actually observed provides a metric of the predictability of evolution. Box 1 provides specific examples of how knowledge of a study system can inform where additional empirical effort is best placed, and Table 1 lists analytical tools that enable prediction. Thus, we propose that focused data collection and analysis can improve prediction of evolution. However, we temper this claim with the caveat that this will not necessarily be an easy task, particularly because the required measurements potentially span different scales of time, space, and biological organization. 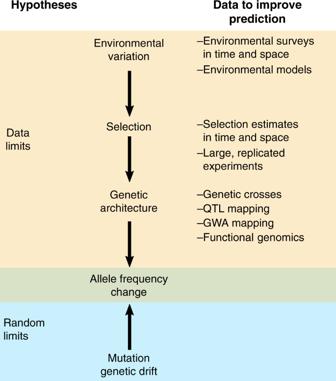Fig. 2: Schematic illustration of two hypotheses for limitations on predicting evolution. This includes depiction of the evolutionary processes involved, and data which might be used to improve prediction. QTL quantitative trait locus, GWA genome wide association. 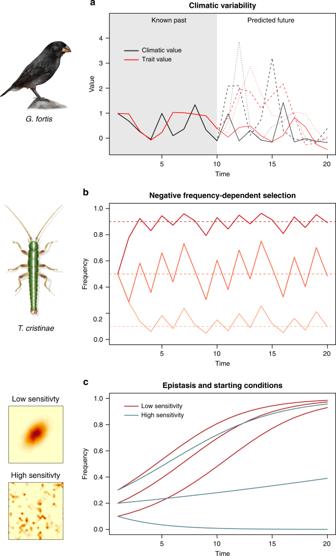Fig. 3: Hypothetical examples of how variation in different factors can limit the predictability of evolution driven by deterministic natural selection. This figure is motivated by empirical systems, but does not depict real data.aUncertainty in climatic variability can limit the predictability of evolution for traits affected by environment-dependent fluctuating selection, such as beak size inG. fortis. Here black lines denote observed (left half) or predicted (right half) climatic values, and red lines denote observed (left half) or predicted (right half) trait values. Multiple possible predictions are shown.bUncertainty in the form of the selection function can limit the predictability of evolution by negative frequency-dependent selection, as is observed for color pattern inT. cristinaestick insects. Possible evolutionary trajectories given three different selection functions (different colored lines) are shown here.cPredictability can also be limited by sensitivity to initial conditions, as occurs on rugged fitness landscapes with considerable epistasis. Two hypothetical fitness landscapes with low (top) and high (bottom) epistasis, and thus sensitivity to initial conditions, are shown (left side; the axes represent genotypes for different loci). Hypothetical evolutionary trajectories from different starting conditions are shown on the right (colored lines). High epistasis promotes different outcomes dependent on initial conditions. Finch and stick insect drawings courtesy of R. Ribas. Table 1 Examples of data types and models that can aid the quantification of uncertainty related to predicting evolution over moderate time scales. Full size table Moreover, many complexities make it difficult to obtain data sufficient for accurate prediction (Fig. 3 ). An example of such a complexity is where mutations interact with one another (i.e., epistasis), rather than having additive effects. Epistasis can cause some genotypic combinations to have much higher fitness than others. Thus, epistasis can cause even adaptive (i.e., non-neutral) evolution to be mediated by historical contingencies in the type and order of mutations that arise [14] , [15] . Specifically, mutations that arise early in evolution can strongly affect which mutations are subsequently viable, making evolution dependent on mutation-order and difficult to predict. For example, mutations that arise early in the evolution of antibiotic resistance effect which subsequent mutations are favored by natural selection [15] . Other interactions, such as those between genes and the environment, are likely to have similar effects for complicating prediction. Fig. 3: Hypothetical examples of how variation in different factors can limit the predictability of evolution driven by deterministic natural selection. This figure is motivated by empirical systems, but does not depict real data. a Uncertainty in climatic variability can limit the predictability of evolution for traits affected by environment-dependent fluctuating selection, such as beak size in G. fortis . Here black lines denote observed (left half) or predicted (right half) climatic values, and red lines denote observed (left half) or predicted (right half) trait values. Multiple possible predictions are shown. b Uncertainty in the form of the selection function can limit the predictability of evolution by negative frequency-dependent selection, as is observed for color pattern in T. cristinae stick insects. Possible evolutionary trajectories given three different selection functions (different colored lines) are shown here. c Predictability can also be limited by sensitivity to initial conditions, as occurs on rugged fitness landscapes with considerable epistasis. Two hypothetical fitness landscapes with low (top) and high (bottom) epistasis, and thus sensitivity to initial conditions, are shown (left side; the axes represent genotypes for different loci). Hypothetical evolutionary trajectories from different starting conditions are shown on the right (colored lines). High epistasis promotes different outcomes dependent on initial conditions. Finch and stick insect drawings courtesy of R. Ribas. Full size image A related issue is sensitivity to initial conditions [11] , which can lead to chaotic dynamics that are deterministic but impossible to predict unless initial conditions are known with extreme precision. An example where this might occur is evolution on highly rugged fitness landscapes, where ruggedness arises due to epistasis. Here, the starting place on a rugged landscape might strongly affect which local fitness peaks are climbed and which valleys are difficult to cross. Although biology may not have a strict counterpart to the Heisenberg uncertainty principle, it is possible that data collection itself alters starting conditions for evolution (e.g., if a human observer scares away predators, this could affect predator-prey dynamics for subsequent evolution). Chaos has received much attention outside of the biological sciences and in the field of ecology, but is not often considered in evolution. All this said, there are also reasons for hope. For example, conceptual and analytical frameworks from the scientific study of complex systems exist to aid prediction of complex phenomena (Table 1 ). Specifically, systems thinking focuses on understanding and predicting how complex networks exhibit emergent properties not shown by individual nodes in the network [16] . In terms of evolution, this involves considering the dynamics of collective networks of genes, populations, and interacting species, rather than trying to use reductionist approaches to understand components in isolation. Because systems approaches apply across scientific disciplines a qualitative analogy can be drawn between the current state of a biological population and the ability to predict its future state based on knowledge of the evolutionary forces operating on it, and the current state of a physical system and the ability to predict its future state based on knowledge of the physical forces acting upon it. In both physics and biology there is the distinction between predictions for individual particles or genes versus the aggregate behavior of many particles (as in statistical thermodynamics) or genes (leading to quantitative genetic breeding values) [17] . In conclusion, although collecting sufficient data for prediction may often represent a formidable challenge, we argue that it is not an insurmountable one. With creative application of emerging technologies and analytical approaches we may improve our ability to predict evolutionary patterns and processes. For example, genomic tools will allow the inference of genetic details such as non-linearities in the genotype-phenotype-fitness map [18] , which can then be incorporated into models to improve prediction. Box 1 provides an example where genomic tools, experiments, and knowledge of genetic and ecological interactions were used to aid prediction of evolution in stick insects. In turn, improved ability to predict evolution may affect our understanding of ecological processes, because to the extent that evolution can be predicted, perhaps so can its ecological consequences for communities and ecosystems [19] . A major avenue for future work is to expand the concepts presented here across broader time scales, where the probability of rare yet consequential events increases. Such longer-term prediction will likely require combining contemporary time series data with deeper phylogenetic patterns, and experimental tests of evolutionary processes. Indeed, progress on this front is exemplified by long-term experimental evolution studies in microbes that demonstrate the effects of rare yet consequential random mutations [20] . Although only further work can reveal the extent to which prediction can be realistically improved, we propose that appreciable progress should be possible in at least some species.